Cyclin B-dependent kinase 1 regulates human TRF1 to modulate the resolution of sister telomeres Cyclin B-Cdk1 is a key mediator of mitotic entry; however, little is known about its role in the separation of sister chromatids. Here we report that upon mitotic entry, Cdk1 specifically phosphorylates threonine 371 of TRF1, a telomere binding protein implicated in the regulation of sister telomere cohesion. Such phosphorylation is removed in late mitosis when Cdk1 activity is inhibited, indicative of a tight regulation of T371 phosphorylation. We show that T371 phosphorylation by Cdk1 keeps TRF1 free of chromatin and this phosphorylation is associated with loss of telomere-bound TRF1 and TIN2, and a reduction in telomere heterochromatin. We find that a phosphomimic mutation at T371 of TRF1 induces telomere deprotection, resulting in telomere loss and the formation of telomere fusions, whereas a non-phosphorylatable substitution of T371 blocks sister telomere resolution, promotes micronuclei formation and impairs cell proliferation. Our work suggests that Cdk1 controls TRF1 association with telomeres to facilitate temporal telomere de-protection, which is essential for sister telomere resolution. Telomeres are specialized heterochromatic structures that function to maintain the integrity and stability of natural chromosome ends in eukaryotic cells. Mammalian telomeric DNA is coated with shelterin, a telomere-specific protein complex composed of TRF1, TRF2, TIN2, Rap1, TPP1 and POT1 (refs 1 , 2 , 3 ). Disruption of shelterin proteins or the telomere heterochromatic state has been shown to induce de-protection of telomeres, resulting in telomere abnormalities such as telomere end-to-end fusions, telomere loss and telomere doublets/fragile telomeres (more than one telomeric signal at a single chromatid end) [4] , [5] , [6] , [7] , [8] , [9] , [10] , [11] . These dysfunctional telomeres are recognized as damaged DNA and are associated with DNA-damage response factors such as γ-H2AX and 53BP1 (refs 7 , 8 , 9 , 12 ). TRF1, a duplex telomeric DNA-binding protein [13] , has a crucial role in telomere metabolism. Knockout of TRF1 leads to early embryonic lethality [14] , indicative of an essential role of TRF1 in development. Conditional deletion of TRF1 induces the formation of fragile telomeres in S phase, a phenomena associated with replication-dependent defects [5] , [8] , suggesting that TRF1 is required to prevent fork stalling, allowing efficient replication of telomeric DNA [8] . Removal of TRF1 from telomeres promotes telomerase-dependent telomere lengthening, whereas overexpression of TRF1 leads to telomere shortening, implying that binding of TRF1 to telomeric DNA negatively regulates the access of telomerase to the ends of telomeres [15] , [16] , [17] . Aside from its role in telomere length maintenance and telomere replication, TRF1 has also been implicated in regulating sister telomere cohesion [18] . Human sister telomeres are fully resolved by the time the cells reach metaphase [19] , [20] , and their resolution has been shown to require the action of tankyrase 1 (ref. 21 ), a poly(ADP-ribose) polymerase known to ribosylate TRF1 (ref. 22 ). Poly(ADP-ribosyl)ation by tankyrase 1 has been reported to release TRF1 from telomeric DNA [22] , rendering TRF1 susceptible to proteosome-dependent degradation [23] , [24] . TRF1 has been shown to physically interact with SA1 (refs 18 , 25 ), a component of the cohesin complex. It has been suggested that the release of TRF1 from telomeres through tankyrase 1-dependent poly(ADP-ribosyl)ation may provide a mechanism to allow for the dissociation of cohesins from telomeres [18] . Depletion of tankyrase 1 has been reported to result in unresolved sister telomeres in mitosis [21] and such a defect can be fully rescued by depletion of SA1 or TIN2 but not TRF1 (ref. 18 ). Thus the role of TRF1 in the separation of sister telomeres has so far been elusive. Cyclin B-dependent kinase 1 (Cdk1) is a key regulator of mitotic entry [26] , [27] and little is known about its role in the separation of sister chromatids. Herein we report that Cdk1 specifically phosphorylates unbound TRF1 at T371 at the time of mitotic entry and that this phosphorylation sequesters TRF1 from binding to telomeres. Such sequestration is associated with loss of telomere-bound TRF1 and TIN2 as well as an accumulation of γ-H2AX, indicating that telomeres undergo temporal de-protection in early mitosis. We show that the lack of T371 phosphorylation by Cdk1 leads to a blockage of sister telomere resolution. Our findings suggest that Cdk1 regulates TRF1 binding to telomeres to facilitate temporal telomere de-protection needed for sister telomere resolution. Cdk1 phosphorylates T371 of TRF1 in early mitosis Mass spectrometry analysis of immunoprecipitated Flag-TRF1 showed threonine 371 of TRF1 to be a candidate phosphorylation site in vivo ( Supplementary Fig. S1a ). We raised an antibody specifically against a TRF1 peptide containing phosphorylated T371 ( Supplementary Fig. S1b,c ) and showed that anti-pT371 antibody predominantly recognized a protein band with an apparent molecular weight indistinguishable from that of endogenous TRF1 ( Fig. 1a ). Depletion of TRF1 resulted in a loss of TRF1 recognized by anti-pT371 antibody ( Fig. 1b ). The antibody also recognized Myc-tagged wild-type TRF1, but not Myc-tagged TRF1 carrying a single amino acid substitution of T371 to either alanine (T371A) or aspartic acid (T371D) ( Fig. 1c ), which was not due to a lack of protein expression ( Fig. 1c ). These results demonstrate that anti-pT371 antibody specifically recognizes phosphorylated T371 of TRF1. 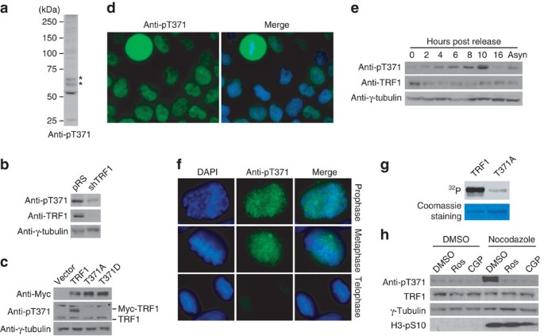Figure 1: T371 of TRF1 is phosphorylated in early mitosis. (a) Western analysis with anti-pT371 antibody. Asterisks indicate non-specific bands that do not respond to shTRF1 knockdown. (b) Western analysis of HeLaII cells depleted for endogenous TRF1. Immunoblotting was performed with anti-pT371 or anti-TRF1 antibody. The γ-tubulin blot was used as a loading control in this experiment and all following westerns shown in this article. (c) Western analysis of various Myc-tagged TRF1 proteins as indicated. Immunoblotting was performed with anti-Myc, anti-pT371 or anti-γ-tubulin antibody. Myc-tagged TRF1 proteins migrate slower than endogenous TRF1. Asterisks indicate non-specific bands that do not respond to shTRF1 knockdown. (d) Indirect immunofluorescence with anti-pT371 antibody on transformed GM637 cells. Original magnification X100. (e) Western analysis of cell extracts from asynchronous HeLaI.2.11 cells (Asyn) or cells released for 0–16 h from a double thymidine block. (f) Indirect immunofluorescence with anti-pT371 antibody on HeLaI.2.11 cells. Original magnification X100. (g)In vitroCdk1 kinase assays. Recombinant cyclin B-Cdk1 was incubated with bacteria-expressed his-tagged wild-type TRF1 or TRF1 mutant T371A in the presence of γ-32P-ATP. (h) Western analysis. HeLaI.2.11 cells were treated with either DMSO or nocodazole, followed by incubation with or without Cdk1 inhibitors Roscovitine (Ros) or CGP74514A (CGP). Immunoblotting was performed with anti-pT371, anti-TRF1, anti-H3pS10 or anti-γ-tubulin antibody. Figure 1: T371 of TRF1 is phosphorylated in early mitosis. ( a ) Western analysis with anti-pT371 antibody. Asterisks indicate non-specific bands that do not respond to shTRF1 knockdown. ( b ) Western analysis of HeLaII cells depleted for endogenous TRF1. Immunoblotting was performed with anti-pT371 or anti-TRF1 antibody. The γ-tubulin blot was used as a loading control in this experiment and all following westerns shown in this article. ( c ) Western analysis of various Myc-tagged TRF1 proteins as indicated. Immunoblotting was performed with anti-Myc, anti-pT371 or anti-γ-tubulin antibody. Myc-tagged TRF1 proteins migrate slower than endogenous TRF1. Asterisks indicate non-specific bands that do not respond to shTRF1 knockdown. ( d ) Indirect immunofluorescence with anti-pT371 antibody on transformed GM637 cells. Original magnification X100. ( e ) Western analysis of cell extracts from asynchronous HeLaI.2.11 cells (Asyn) or cells released for 0–16 h from a double thymidine block. ( f ) Indirect immunofluorescence with anti-pT371 antibody on HeLaI.2.11 cells. Original magnification X100. ( g ) In vitro Cdk1 kinase assays. Recombinant cyclin B-Cdk1 was incubated with bacteria-expressed his-tagged wild-type TRF1 or TRF1 mutant T371A in the presence of γ- 32 P-ATP. ( h ) Western analysis. HeLaI.2.11 cells were treated with either DMSO or nocodazole, followed by incubation with or without Cdk1 inhibitors Roscovitine (Ros) or CGP74514A (CGP). Immunoblotting was performed with anti-pT371, anti-TRF1, anti-H3pS10 or anti-γ-tubulin antibody. Full size image Analysis of indirect immunofluorescence showed that anti-pT371 antibody stained mitotic cells much more intensely than interphase cells ( Fig. 1d ; Supplementary Fig. S2 ). Western analysis also showed an increase in T371 phosphorylation in cells 10 h post release from a double thymidine block ( Fig. 1e ). Previously, we have shown that cells entered mitosis 10 h post release [28] . Examination of the sub-stages of mitosis showed that T371 phosphorylation was specifically upregulated in prophase and metaphase and such upregulation was completely abolished when cells entered telophase ( Fig. 1f ; Supplementary Fig. S2 ). These results show that T371 phosphorylation is cell-cycle regulated, peaking in early mitosis. T371 (T 371 PEK) matches the consensus sequence for Cdk1, a cyclin-dependent kinase essential for the G2/M transition. An alanine substitution of T371 drastically abrogated TRF1 phosphorylation by Cdk1 in vitro ( Fig. 1g ), consistent with previous findings [29] . Treatment with Cdk1 inhibitors (CGP74514A or Roscovitine) completely abolished the increase of TRF1 phosphorylation associated with the nocodazole arrest, but it had no effect on phosphorylation of serine 10 of H3, a substrate of Aurora B ( Fig. 1h ), suggesting that Cdk1 is the main kinase responsible for T371 phosphorylation in early mitosis. T371 phosphorylation by Cdk1 keeps TRF1 free of chromatin Pre-incubation of TRF1 with telomeric DNA completely abolished TRF1 phosphorylation by Cdk1 ( Fig. 2a ). The inhibitory effect of telomeric DNA on TRF1 phosphorylation by Cdk1 was not observed with a TRF1 mutant (TRF1-R425V) ( Fig. 2a ), which has been previously reported to be unable to bind to telomeric DNA [30] . Furthermore, pre-incubation with telomeric DNA did not inhibit phosphorylation of H1 by Cdk1 ( Fig. 2a ). These results suggest that Cdk1 specifically phosphorylates unbound TRF1 and that when bound to telomeric DNA, TRF1 may become inaccessible for phosphorylation by Cdk1, perhaps owing to a conformational change. 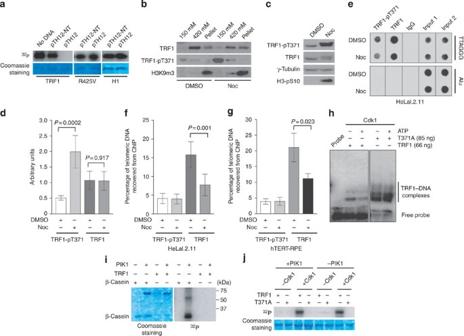Figure 2: Cdk1 specifically phosphorylates unbound TRF1 and this phosphorylation keeps TRF1 free of chromatin. (a) Two micrograms of recombinant wild-type TRF1, mutant TRF1-R425V or H1 was pre-incubated with no DNA or 5 μg of pTH12-NT (non-telomeric DNA) or pTH12 (telomeric DNA), followed by Cdk1 kinase assays. (b) Differential salt extraction of chromatin on HeLaI.2.11 cells treated with DMSO or nocodazole (Noc). (c) Western analysis. (d) Quantification of total TRF1 and phosphorylated TRF1 from (c). The signals from the western blots were quantified with densitometry. The level of total TRF1 and phosphorylated TRF1 are represented in arbitrary units after their signals were normalized relative to those of γ-tubulin. A Student's two-tailedt-test was used to derive allPvalues. Standard deviations from three independent experiments are indicated. (e) Dot blots of ChIPs with anti-pT371 or anti-TRF1 antibody. HeLaI.2.11 cells were treated with DMSO or nocodazole. Anti-IgG antibody was used as a negative control in this experiment and all the following ChIPs shown in this article. (f) Quantification of ChIPs from (e). ImageQuant analysis was used for quantification in this experiment and all the following ChIPs shown in this article. ThePvalue was calculated using a Student's two-tailedt-test. Standard deviation are derived from at least four independent experiments. (g) Quantification of ChIPs with anti-pT371 or anti-TRF1 antibody from hTERT-RPE cell extracts. ThePvalue was calculated using a Student's two-tailedt-test. Standard deviation from three independent experiments are indicated. (h) DNA binding assays. Before gel shift assays, recombinant wild-type TRF1 (66 ng) or T371A (85 ng) was incubated with BSA (1 μg) and Cdk1 with or without 5 mM cold ATP. BSA was used as a competitor for the non-specific activity of Cdk1. (i) Recombinant Plk1 was incubated with recombinant wild-type TRF1 or β-casein in the presence of γ-32P-ATP. Recombinant TRF1 comigrates with Plk1 on an 8% SDS–polyacrylamide gel. (j) Sequential kinase assays. Recombinant wild-type TRF1 or TRF1-T371A was incubated with cold ATP with or without Cdk1, followed by addition of γ-32P-ATP in the presence of Plk1 or no Plk1 as indicated above the lanes. Figure 2: Cdk1 specifically phosphorylates unbound TRF1 and this phosphorylation keeps TRF1 free of chromatin. ( a ) Two micrograms of recombinant wild-type TRF1, mutant TRF1-R425V or H1 was pre-incubated with no DNA or 5 μg of pTH12-NT (non-telomeric DNA) or pTH12 (telomeric DNA), followed by Cdk1 kinase assays. ( b ) Differential salt extraction of chromatin on HeLaI.2.11 cells treated with DMSO or nocodazole (Noc). ( c ) Western analysis. ( d ) Quantification of total TRF1 and phosphorylated TRF1 from ( c ). The signals from the western blots were quantified with densitometry. The level of total TRF1 and phosphorylated TRF1 are represented in arbitrary units after their signals were normalized relative to those of γ-tubulin. A Student's two-tailed t -test was used to derive all P values. Standard deviations from three independent experiments are indicated. ( e ) Dot blots of ChIPs with anti-pT371 or anti-TRF1 antibody. HeLaI.2.11 cells were treated with DMSO or nocodazole. Anti-IgG antibody was used as a negative control in this experiment and all the following ChIPs shown in this article. ( f ) Quantification of ChIPs from ( e ). ImageQuant analysis was used for quantification in this experiment and all the following ChIPs shown in this article. The P value was calculated using a Student's two-tailed t -test. Standard deviation are derived from at least four independent experiments. ( g ) Quantification of ChIPs with anti-pT371 or anti-TRF1 antibody from hTERT-RPE cell extracts. The P value was calculated using a Student's two-tailed t -test. Standard deviation from three independent experiments are indicated. ( h ) DNA binding assays. Before gel shift assays, recombinant wild-type TRF1 (66 ng) or T371A (85 ng) was incubated with BSA (1 μg) and Cdk1 with or without 5 mM cold ATP. BSA was used as a competitor for the non-specific activity of Cdk1. ( i ) Recombinant Plk1 was incubated with recombinant wild-type TRF1 or β-casein in the presence of γ- 32 P-ATP. Recombinant TRF1 comigrates with Plk1 on an 8% SDS–polyacrylamide gel. ( j ) Sequential kinase assays. Recombinant wild-type TRF1 or TRF1-T371A was incubated with cold ATP with or without Cdk1, followed by addition of γ- 32 P-ATP in the presence of Plk1 or no Plk1 as indicated above the lanes. Full size image Analysis of differential salt extraction of chromatin showed that TRF1 was chromatin-bound (420 mM KCl fraction) and very little TRF1 was detected in the chromatin-free fraction (150 mM KCl) in DMSO-treated cells ( Fig. 2b ), consistent with previous findings [31] . However, on nocodazole treatment, we observed a reduction in the amount of chromatin-bound TRF1 and the appearance of chromatin-free TRF1, which coincided with a sharp increase in T371 phosphorylation that was predominantly (if not all) chromatin free ( Fig. 2b ). Nocodazole treatment resulted in an enrichment of mitotic cells ( Supplementary Fig. S3a ; Fig. 2c ) and no release of the heterochromatic mark H3K9m3 from chromatin was observed in mitosis ( Fig. 2b ; Supplementary Fig. S3b ). The reduction of chromatin-bound TRF1 in nocodazole-treated cells was also observed in our chromatin immunoprecipitation (ChIP) analysis. Although nocodazole treatment did not affect the level of total TRF1 ( Fig. 2c,d ), it resulted in at least a 50% decrease in telomeric association of total TRF1 ( Fig. 2e,f ). Such a decrease was also seen in nocodazole-treated hTERT-immortalized normal cells (hTERT-RPE) ( Fig. 2g ). Nocodazole treatment led to a fourfold increase in the level of T371 phosphorylation ( Fig. 2c,d ), and yet no increase in the association of phosphorylated TRF1 with telomeric DNA was observed ( Fig. 2e,f ). These results, together with our earlier finding that most of anti-pT371 staining in mitotic cells did not overlap with DAPI staining, suggest that T371 phosphorylation by Cdk1 sequesters TRF1 from associating with telomere chromatin. Consistent with our in vivo findings, pre-phosphorylation of the recombinant wild-type TRF1 by Cdk1 resulted in a reduction in TRF1 binding to telomeric DNA, whereas telomeric DNA binding of TRF1-T371A was not impaired by pretreatment with Cdk1 and ATP ( Fig. 2h ). BSA was included in the gel-shift assays to minimize the non-specific stimulation of the in vitro DNA binding activity of TRF1 by Cdk1 and such non-specific stimulation has also been observed for a number of other proteins [13] , [22] . These results suggest that T371 phosphorylation by Cdk1 negatively regulates TRF1 binding to telomeric DNA. Previously it has been suggested that phosphorylation of T344 and T371 by Cdk1 serves as a docking site for TRF1 phosphorylation by Plk1 (ref. 29 ), which has been reported to stimulate TRF1 binding to telomeric DNA [29] . However, we did not observe any TRF1 phosphorylation by Plk1 despite the fact Plk1 readily phosphorylated β-Casein ( Fig. 2i ), a positive control for Plk1. Furthermore, we failed to detect any TRF1 phosphorylation by Plk1 even when TRF1 was preincubated with Cdk1 and cold ATP ( Fig. 2j ). The phosphorylation signal observed in the lane containing both Cdk1 and Plk1 was likely due to the action of Cdk1 alone, because a similar level of TRF1 phosphorylation was also detected in the lane containing only Cdk1 and no Plk1 ( Fig. 2j ). Such signal was completely absent when TRF1-T371A was used in the reaction ( Fig. 2j ). Although we cannot rule out the possibility that the difference in the source of recombinant proteins used might have contributed to the lack of TRF1 phosphorylation by Plk1, our finding that Plk1 can readily phosphorylate β-Casein but not TRF1 suggests that the lack of TRF1 phosphorylation signal is unlikely due to Plk1 activity. Our findings that T371 phosphorylation by Cdk1 negatively regulates TRF1 interaction with telomeric DNA both in vivo and in vitro , along with the lack of a detectable stimulation of Plk1-dependent TRF1 phosphorylation by Cdk1, strongly argue against the previously suggested possibility that T371 phosphorylation by Cdk1 may serve as a positive regulator of TRF1 binding [29] . Dephosphorylation of T371 allows TRF1 binding to telomeres To examine whether the loss of T371 phosphorylation in telophase cells ( Fig. 1f ) might be due to phosphatase activity, we arrested HeLaI.2.11 cells in nocodazole and then released them into media containing either DMSO or okadaic acid, the latter being a potent phosphatase inhibitor [32] . Cells remained in mitosis 30-min post release from the nocodazole arrest, but they started to exit mitosis 90-min post release ( Fig. 3a ). T371 phosphorylation persisted in okadaic acid-treated cells but was diminished in DMSO-treated cells 90-min post release ( Fig. 3b ). The level of total TRF1 was not affected by treatment with okadaic acid ( Fig. 3b ). These results suggest that T371 undergoes dephosphorylation in late mitosis. 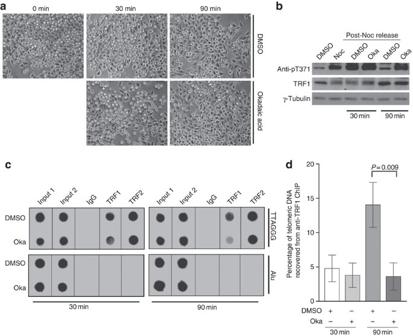Figure 3: T371 of TRF1 is dephosphorylated in late mitosis and this dephosphorylation allows the re-association of TRF1 with telomeric DNA. (a) Live cell images for HeLaI.2.11 cells released from a nocodazole arrest into fresh media containing either DMSO or okadaic acid (Oka) (1 μM) for 0–90 min. Original magnification X20. (b) Western analysis performed with anti-pT371, anti-TRF1 or anti-γ-tubulin antibody. (c) Dot blots of ChIPs performed with anti-TRF1 or anti-TRF2 antibody. Nocodazole-arrested HeLaI.2.11 cells were released into fresh media containing either DMSO or okadaic acid for either 30 or 90 min. (d) Quantification of anti-TRF1 ChIPs from (c). ThePvalue was calculated using a Student's two-tailedt-test. Standard deviations derived from at least three independent experiments are indicated. Figure 3: T371 of TRF1 is dephosphorylated in late mitosis and this dephosphorylation allows the re-association of TRF1 with telomeric DNA. ( a ) Live cell images for HeLaI.2.11 cells released from a nocodazole arrest into fresh media containing either DMSO or okadaic acid (Oka) (1 μM) for 0–90 min. Original magnification X20. ( b ) Western analysis performed with anti-pT371, anti-TRF1 or anti-γ-tubulin antibody. ( c ) Dot blots of ChIPs performed with anti-TRF1 or anti-TRF2 antibody. Nocodazole-arrested HeLaI.2.11 cells were released into fresh media containing either DMSO or okadaic acid for either 30 or 90 min. ( d ) Quantification of anti-TRF1 ChIPs from ( c ). The P value was calculated using a Student's two-tailed t -test. Standard deviations derived from at least three independent experiments are indicated. Full size image Anti-TRF1 ChIP analysis showed that 30-min post release, telomeric association of TRF1 in cells grown in DMSO-containing media was indistinguishable from that in cells grown in okadaic acid-containing media ( Fig. 3c,d ). However, 90-min post release, cells grown in DMSO-containing media exhibited a 3.9-fold increase in TRF1 association with telomeric DNA compared with cells cultured in okadaic acid-containing media ( Fig. 3c,d ). As TRF1 remained phosphorylated at T371 30-min post release, T371 was dephosphorylated in cells grown in DMSO-containing media by 90 min post release ( Fig. 3b ). Treatment with okadaic acid did not affect the total level of TRF1 ( Fig. 3b ), nor did it affect telomeric association of TRF2 ( Fig. 3c ). These results suggest that TRF1 is re-associated with telomeric DNA in late mitosis as a result of T371 dephosphorylation. Telomeres are recognized as damaged DNA in early mitosis To investigate whether the loss of telomere-bound TRF1 in early mitosis might affect telomeric association of other shelterin proteins, we arrested cells with nocodazole and performed ChIPs with anti-TIN2 or anti-TRF2 antibody. Nocodazole treatment caused a 35% reduction in telomeric association of TIN2 ( Fig. 4a,b ), but had no effect on telomeric association of TRF2 ( Fig. 4a,b ). The total level of TIN2 or TRF2 was not affected by nocodazole treatment ( Fig. 4c ). 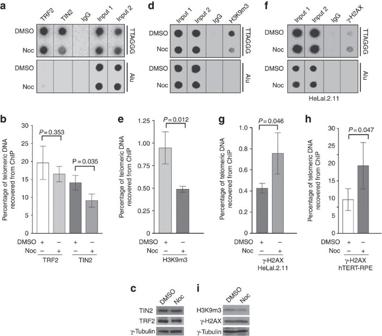Figure 4: Nocodazole arrest results in loss of TIN2 and the heterochromatic mark at telomeres and an accumulation of γ-H2AX at telomeres. (a) Dot blots of anti-TIN2 and anti-TRF2 ChIPs from HeLaI.2.11 cells treated with either DMSO or nocodazole. (b) Quantification of anti-TRF2 and anti-TIN2 ChIPs from (a). ThePvalue was calculated using a Student's two-tailedt-test. Standard deviations from three independent experiments are indicated. (c) Western analysis with anti-TIN2, anti-TRF2 or anti-γ-tubulin antibody. (d) Dot blots of anti-H3K9m3 ChIPs from HeLaI.2.11 cells treated with either DMSO or nocodazole. (e) Quantification of anti-H3K9m3 ChIPs. ThePvalue was calculated using a Student's two-tailedt-test. Standard deviations from three independent experiments are indicated. (f) Dot blots of anti-γ-H2AX ChIPs from HeLaI.2.11 cells treated with either DMSO or nocodazole. (g) Quantification of anti-γ-H2AX ChIPs from (f). ThePvalue was calculated using a Student's two-tailedt-test. Standard deviations from three independent experiments are indicated. (h) Quantification of anti-γ-H2AX ChIPs for hTERT-RPE cells. ThePvalue was calculated using a Student's two-tailedt-test. Standard deviations from three independent experiments are indicated. (i) Western analysis with anti-H3K9m3, anti-γ-H2AX or anti-γ-tubulin antibody. Figure 4: Nocodazole arrest results in loss of TIN2 and the heterochromatic mark at telomeres and an accumulation of γ-H2AX at telomeres. ( a ) Dot blots of anti-TIN2 and anti-TRF2 ChIPs from HeLaI.2.11 cells treated with either DMSO or nocodazole. ( b ) Quantification of anti-TRF2 and anti-TIN2 ChIPs from ( a ). The P value was calculated using a Student's two-tailed t -test. Standard deviations from three independent experiments are indicated. ( c ) Western analysis with anti-TIN2, anti-TRF2 or anti-γ-tubulin antibody. ( d ) Dot blots of anti-H3K9m3 ChIPs from HeLaI.2.11 cells treated with either DMSO or nocodazole. ( e ) Quantification of anti-H3K9m3 ChIPs. The P value was calculated using a Student's two-tailed t -test. Standard deviations from three independent experiments are indicated. ( f ) Dot blots of anti-γ-H2AX ChIPs from HeLaI.2.11 cells treated with either DMSO or nocodazole. ( g ) Quantification of anti-γ-H2AX ChIPs from ( f ). The P value was calculated using a Student's two-tailed t -test. Standard deviations from three independent experiments are indicated. ( h ) Quantification of anti-γ-H2AX ChIPs for hTERT-RPE cells. The P value was calculated using a Student's two-tailed t -test. Standard deviations from three independent experiments are indicated. ( i ) Western analysis with anti-H3K9m3, anti-γ-H2AX or anti-γ-tubulin antibody. Full size image Anti-H3K9m3 ChIP analysis showed that nocodazole treatment resulted in a 50% reduction in telomeric association of the heterochromatic mark H3K9 trimethylation ( Fig. 4d,e ) in HeLaI.2.11 cells. Along with the loss of telomere-bound H3K9m3, we also observed a substantial increase in γ-H2AX association with telomeres in both HeLaI.2.11 and hTERT-RPE cells treated with nocodazole ( Fig. 4f,g,h ), indicative of telomere uncapping in early mitosis. The reduction in the amount of H3K9m3 at telomeres is unlikely due to a change in the total level of trimethylated H3K9 ( Fig. 4i ) or its ability to associate with chromatin in mitosis ( Fig. 2b ; Supplementary Fig. S3b ). Our finding that γ-H2AX was accumulated at telomeres in nocodazole-treated hTERT-RPE cells suggests that the observed telomere uncapping in early mitosis is unlikely to be solely the result of escaped damage from the previous G2 due to a non-functional p53 pathway as reported [33] . These results suggest that telomeres lose their heterochromatic state and are temporally recognized as damaged DNA in early mitosis. T371 phosphorylation protects unbound TRF1 from degradation To examine whether T371 phosphorylation might be involved in regulating TRF1 stability, we subjected nocodazole-treated HeLa cells to cycloheximide experiments in the presence of okadaic acid, which was used to prevent dephosphorylation of TRF1. Phosphorylated (pT371)TRF1 showed a slower rate of degradation than total TRF1 ( Fig. 5a,b ). Consistent with this finding, the phosphomimic TRF1-T371D mutant was significantly more stable than wild-type TRF1 ( Fig. 5c,d ). At 8 h post-cycloheximide chase, about 61% of Myc-tagged wild-type TRF1 was degraded, whereas no degradation was observed for Myc-tagged TRF1-T371D ( Fig. 5d ). These results suggest that T371 phosphorylation by Cdk1 protects the pool of unbound TRF1 from being targeted for degradation. 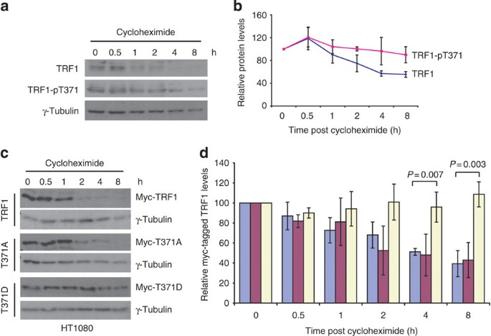Figure 5: Phosphorylation of T371 protects TRF1 from being targeted for degradation. (a) Cycloheximide chase experiments. Nocodazole-arrested HeLaI.2.11 cells were treated with cycloheximide (100 μg ml-1) in the presence of 1 μM okadaic acid for the indicated times. Okadaic acid was used to prevent dephosphorylation of T371. Immunoblotting was performed with anti-TRF1, anti-pT371 or anti-γ-tubulin antibody. (b) Quantification of total TRF1 and phosphorylated (pT371)TRF1 from (a). The signals from the western blots were quantified with densitometry. The level of total TRF1 or phosphorylated (pT371)TRF1 is represented in arbitrary units after their signals were normalized relative to those of γ-tubulin. Standard deviations from three independent experiments are indicated. (c) Cycloheximide chase experiments. HT1080 cells expressing Myc-TRF1, Myc-TRF1-T371A or Myc-TRF1-T371D were treated with 100 μg ml-1cycloheximide for the indicated times, followed by immunoblotting of the lysates with anti-Myc or anti-γ-tubulin antibody. (d) Quantification of Myc-tagged wild-type TRF1 (blue bars), Myc-tagged TRF1-T371A (purple bars) and Myc-tagged TRF1-T371D (light yellow bars) from (c). Quantification was performed as described in (b). AllPvalues were calculated using a Student's two-tailedt-test. Standard deviations from three independent experiments are indicated. Figure 5: Phosphorylation of T371 protects TRF1 from being targeted for degradation. ( a ) Cycloheximide chase experiments. Nocodazole-arrested HeLaI.2.11 cells were treated with cycloheximide (100 μg ml -1 ) in the presence of 1 μM okadaic acid for the indicated times. Okadaic acid was used to prevent dephosphorylation of T371. Immunoblotting was performed with anti-TRF1, anti-pT371 or anti-γ-tubulin antibody. ( b ) Quantification of total TRF1 and phosphorylated (pT371)TRF1 from ( a ). The signals from the western blots were quantified with densitometry. The level of total TRF1 or phosphorylated (pT371)TRF1 is represented in arbitrary units after their signals were normalized relative to those of γ-tubulin. Standard deviations from three independent experiments are indicated. ( c ) Cycloheximide chase experiments. HT1080 cells expressing Myc-TRF1, Myc-TRF1-T371A or Myc-TRF1-T371D were treated with 100 μg ml -1 cycloheximide for the indicated times, followed by immunoblotting of the lysates with anti-Myc or anti-γ-tubulin antibody. ( d ) Quantification of Myc-tagged wild-type TRF1 (blue bars), Myc-tagged TRF1-T371A (purple bars) and Myc-tagged TRF1-T371D (light yellow bars) from ( c ). Quantification was performed as described in ( b ). All P values were calculated using a Student's two-tailed t -test. Standard deviations from three independent experiments are indicated. Full size image Persistent T371 phosphorylation promotes telomere uncapping TRF1-depleted HeLaII cells were infected with retrovirus expressing the vector alone, Myc-tagged wild-type TRF1 (resistant to shTRF1 due to engineered silent mutations), Myc-tagged TRF1-T371A or Myc-tagged TRF1-T371D, giving rise to four stable cell lines (shTRF1-vector, shTRF1-TRF1, shTRF1-T371A, shTRF1-T371D). We chose to use TRF1-depleted cells for analysis of TRF1 mutants to minimize the interference from endogenous TRF1. ChIP analysis showed that Myc-TRF1-T371D exhibited a 41% decrease in its association with telomeric DNA compared with wild-type TRF1, whereas binding of Myc-TRF1-T371A to telomeric DNA was similar to that of wild-type TRF1 ( Fig. 6a,b ). Expression of TRF1 mutants was indistinguishable from that of wild-type TRF1 ( Fig. 6c ). The impaired ability of the phosphomimic mutant to associate with telomeric DNA was also demonstrated through in vitro gel-shift assays using bacteria-expressed recombinant TRF1 proteins ( Fig. 6d,e ). Furthermore, analysis of differential salt extraction showed that the amount of chromatin-bound Myc-TRF1-T371D was severely reduced compared with that of chromatin-bound wild-type TRF1 or Myc-TRF1-T371A ( Fig. 6f ). The amount of chromatin-bound TRF2 was not reduced in Myc-TRF1-T371D-expressing cells ( Fig. 6f ), suggesting that the loss of chromatin-bound Myc-TRF1-T371D was specific. We also observed a slight decrease in the amount of chromatin-bound TIN2 in Myc-TRF1-T371D-expressing cells ( Fig. 6f ), consistent with our earlier finding that T371 phosphorylation in mitosis was associated with loss of TIN2 at telomeres ( Fig. 4a,b ). Overexpression of TRF1-T371D resulted in a 46% loss of trimethylated H3K9 at telomeres compared with wild-type TRF1 although overexpression of TRF1-T371A had little impact on H3K9m3 at telomeres ( Fig. 6g,h ). Expression of TRF1 mutants did not affect the total level of H3K9 trimethylation ( Fig. 6i ). These results altogether suggest that T371D mimics T371 phosphorylation and that persistent phosphorylation of T371 induces loss of telomere heterochromatin. 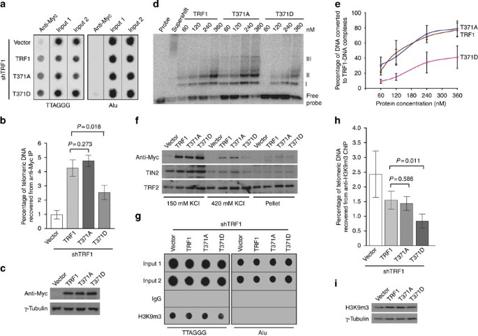Figure 6: Phosphomimic mutation at T371 (T371D) impairs TRF1 interaction with telomeres and promotes loss of telomere heterochromatin. (a) Dot blots of anti-Myc ChIPs from TRF1-depleted HeLaII cells expressing various constructs as indicated on the left. (b) Quantification of anti-Myc ChIPs from (a). ThePvalues were calculated using a Student's two-tailedt-test. Standard deviations from three independent experiments are indicated. (c) Western analysis of Myc-tagged TRF1 proteins. (d)In vitrogel shift assays. Bacteria-derived recombinant TRF1 proteins were used in the gel-shift assays as indicated above the lanes. The positions of three TRF1-containing complexes (I, II and III) are indicated on the right. All TRF1-containing complexes can be supershifted by anti-TRF1 antibody. The concentrations of recombinant TRF1 used were indicated above the lanes. (e) Quantification of percentage of total DNA converted to TRF1–DNA complexes. Standard deviations for TRF1 mutants (T371A and T371D) were derived from three independent experiments, whereas standard deviations for wild-type TRF1 were derived from at least two independent experiments. (f) Differential salt extraction of chromatin on TRF1-depleted cells expressing various constructs as indicated above the lanes. (g) Dot blots of anti-H3K9m3 ChIPs from TRF1-depleted HeLaII cells expressing various constructs as indicated. (h) Quantification of anti-H3K9m3 ChIPs. ThePvalues were calculated using a Student's two-tailedt-test. Standard deviations derived from four independent experiments are indicated. (i) Western analysis of H3K9m3 expression. Figure 6: Phosphomimic mutation at T371 (T371D) impairs TRF1 interaction with telomeres and promotes loss of telomere heterochromatin. ( a ) Dot blots of anti-Myc ChIPs from TRF1-depleted HeLaII cells expressing various constructs as indicated on the left. ( b ) Quantification of anti-Myc ChIPs from ( a ). The P values were calculated using a Student's two-tailed t -test. Standard deviations from three independent experiments are indicated. ( c ) Western analysis of Myc-tagged TRF1 proteins. ( d ) In vitro gel shift assays. Bacteria-derived recombinant TRF1 proteins were used in the gel-shift assays as indicated above the lanes. The positions of three TRF1-containing complexes (I, II and III) are indicated on the right. All TRF1-containing complexes can be supershifted by anti-TRF1 antibody. The concentrations of recombinant TRF1 used were indicated above the lanes. ( e ) Quantification of percentage of total DNA converted to TRF1–DNA complexes. Standard deviations for TRF1 mutants (T371A and T371D) were derived from three independent experiments, whereas standard deviations for wild-type TRF1 were derived from at least two independent experiments. ( f ) Differential salt extraction of chromatin on TRF1-depleted cells expressing various constructs as indicated above the lanes. ( g ) Dot blots of anti-H3K9m3 ChIPs from TRF1-depleted HeLaII cells expressing various constructs as indicated. ( h ) Quantification of anti-H3K9m3 ChIPs. The P values were calculated using a Student's two-tailed t -test. Standard deviations derived from four independent experiments are indicated. ( i ) Western analysis of H3K9m3 expression. Full size image Overexpression of TRF1-T371D promoted the formation of lagging chromosomes and anaphase bridges ( Supplementary Fig. S4 ), the latter of which suggests the formation of telomere fusions. Depletion of TRF1 did not promote the formation of telomere-containing extra-chromosomal DNA but resulted in the induction of telomere doublets, telomere loss and sister telomere fusions ( Supplementary Fig. S5 ), which is consistent with previous findings [5] , [8] . Overexpression of wild-type TRF1 was able to suppress the formation of all these abnormalities in TRF1-depleted cells ( Fig. 7a–f ). Introduction of either TRF1-T371A or TRF1-T371D into TRF1-depleted cells suppressed the formation of telomere doublets, similar to that of wild-type TRF1 ( Fig. 7b ; Supplementary Fig. S6 ). Aphidicolin, an inhibitor of DNA replication, has been shown to induce telomere doublets, which are thought to arise from a defect in telomere replication [5] , [8] . We observed a striking increase in telomere doublets in TRF1-depleted cells on treatment with aphidicolin ( Fig. 7c ), which is consistent with a previous report [8] that the effect of aphidicolin was additive with loss of TRF1. Such an increase was not observed in TRF1-depleted cells expressing wild-type TRF1, TRF1-T371A or TRF1-T371D ( Fig. 7c ). These results suggest that T371 may not be required for the function of TRF1 in telomere replication. 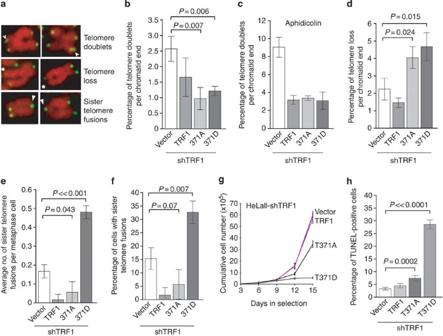Figure 7: Overexpression of TRF1-T371D promotes telomere uncapping and results in induction of apoptosis. (a) Images of metaphase chromosomes depicting telomere abnormalities. Metaphase chromosomes were stained with DAPI and false-colored in red. Telomeric DNA was detected by FISH using a FITC-conjugated (CCCTAA)3-containing PNA probe in green. Open arrows: telomere doublets. Asterisks represent telomere loss, whereas filled arrows indicate sister telomere fusions. Original magnification X100. (b) Quantification of telomere doublets from TRF1-depleted cells expressing indicated constructs. For each cell line, a total of 3,486–4,696 chromosomes from 52 to 71 metaphase cells were scored in a blind manner for the presence of telomere doublets in (b,c) as well as telomere loss in (d) and sister telomere fusions in (e,f). AllPvalues shown in (b–f,h) were calculated using a Student's two-tailedt-test. Standard deviations derived from three independent experiments are indicated. (c) Quantification of telomere doublets from aphidicolin-treated cells. (d) Quantification of telomere loss from TRF1-depleted cells expressing indicated constructs. Telomere loss refers to chromatids without a detectable telomere signal. The total number of chromatid ends without a detectable telomere signal was divided by the total number of chromatid ends scored, giving rise to the percentage of telomere loss per chromatid end. (e) Quantification of average number of sister telomere fusions per metaphase cell from TRF1-depleted cells expressing indicated constructs. (f) Quantification of percentage of cells with sister telomere fusions from TRF1-depleted cells expressing indicated constructs. (g) Proliferation assays of TRF1-depleted cells expressing various constructs as indicated. Standard deviations from three independent experiments are indicated. (h) Quantification of TUNEL assays. Scoring of TRF1-depleted HeLaII cells expressing various constructs as indicated was done in a blind manner. A total of 1,000 cells from each of four independent experiments were scored. Standard deviations are derived from four independent experiments. Figure 7: Overexpression of TRF1-T371D promotes telomere uncapping and results in induction of apoptosis. ( a ) Images of metaphase chromosomes depicting telomere abnormalities. Metaphase chromosomes were stained with DAPI and false-colored in red. Telomeric DNA was detected by FISH using a FITC-conjugated (CCCTAA) 3 -containing PNA probe in green. Open arrows: telomere doublets. Asterisks represent telomere loss, whereas filled arrows indicate sister telomere fusions. Original magnification X100. ( b ) Quantification of telomere doublets from TRF1-depleted cells expressing indicated constructs. For each cell line, a total of 3,486–4,696 chromosomes from 52 to 71 metaphase cells were scored in a blind manner for the presence of telomere doublets in ( b , c ) as well as telomere loss in ( d ) and sister telomere fusions in ( e , f ). All P values shown in ( b – f , h ) were calculated using a Student's two-tailed t -test. Standard deviations derived from three independent experiments are indicated. ( c ) Quantification of telomere doublets from aphidicolin-treated cells. ( d ) Quantification of telomere loss from TRF1-depleted cells expressing indicated constructs. Telomere loss refers to chromatids without a detectable telomere signal. The total number of chromatid ends without a detectable telomere signal was divided by the total number of chromatid ends scored, giving rise to the percentage of telomere loss per chromatid end. ( e ) Quantification of average number of sister telomere fusions per metaphase cell from TRF1-depleted cells expressing indicated constructs. ( f ) Quantification of percentage of cells with sister telomere fusions from TRF1-depleted cells expressing indicated constructs. ( g ) Proliferation assays of TRF1-depleted cells expressing various constructs as indicated. Standard deviations from three independent experiments are indicated. ( h ) Quantification of TUNEL assays. Scoring of TRF1-depleted HeLaII cells expressing various constructs as indicated was done in a blind manner. A total of 1,000 cells from each of four independent experiments were scored. Standard deviations are derived from four independent experiments. Full size image In contrast to the phenotype of telomere doublets, overexpresion of either TRF1-T371A or TRF1-T371D further promoted telomere loss in TRF1-depleted cells ( Fig. 7d ; Supplementary Fig. S6 ). Compared with the vector alone in TRF1-depleted cells, an increase of 1.8- and 2.1-fold in telomere loss was observed in cells expressing either TRF1-T371A or TRF1-T371D, respectively ( Fig. 7d ). In addition, overexpression of TRF1-T371D further induced the formation of sister telomere fusions in TRF1-depleted cells ( Fig. 7e,f ; Supplementary Fig. S6 ). It is unlikely that these fusions were mistaken for chromosomes that are missing a detectable telomere signal on one sister chromatid, as they were suppressed in TRF1-T371A-expressing cells that exhibited an accumulation of telomere loss ( Fig. 7d ). Compared with the vector alone, the average number of sister telomere fusions nearly tripled in TRF1-T371D-expressing cells ( Fig. 7e ), suggesting that persistent phosphorylation of T371 leads to telomere uncapping. Cell proliferation assays showed that cells overexpressing TRF1-T371D failed to proliferate compared with the vector-expressing cells ( Fig. 7g ). Such a failure was associated with a high rate of apoptosis as shown by TdT-mediated dUTP nick end labelling (TUNEL) assays ( Fig. 7h ; Supplementary Fig. S7 ). Compared with the vector alone, a sharp increase of 8.7-fold in cell death was observed in TRF1-depleted cells expressing TRF1-T371D ( Fig. 7h ). These results suggest that TRF1-T371D-induced telomere uncapping promotes the induction of apoptosis. Lack of T371 phosphorylation blocks sister telomere resolution Anti-Myc ChIP analysis showed that in nocodazole-arrested cells, TRF1-T371A exhibited a 1.9-fold increase in its association with telomeric DNA compared with wild-type TRF1 ( Fig. 8a,b ), whereas the level of Myc-TRF1-T371A was indistinguishable from that of Myc-tagged wild-type TRF1 ( Fig. 8c ), suggesting that the lack of T371 phosphorylation leads to an increase in TRF1 binding to telomeric DNA in early mitosis. 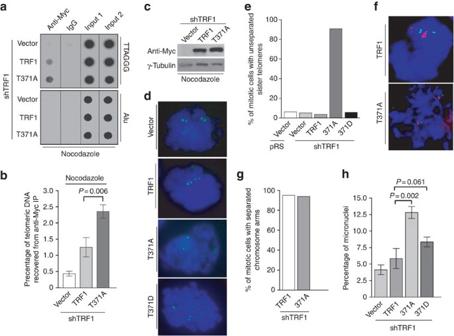Figure 8: Lack of phosphorylation at T371 leads to near complete blockage of the resolution of sister telomeres. (a) Dot blots of anti-Myc ChIPs. TRF1-depleted HeLaII cells, expressing various constructs as indicated, were treated with nocodazole before ChIP analysis. (b) Quantification of anti-Myc ChIPs. Standard deviations derived from three independent experiments are indicated. (c) Western analysis of Myc-tagged TRF1 expression. (d) Chromosome-specific FISH with a FITC-labelled subtelomere specific probe (16pter; Cytocell) in green. DNA was stained with DAPI shown in blue. Original magnification X100. (e) Quantification of metaphase cells carrying unresolved sister telomeres. Metaphase cells carrying two sets of a green doublet were scored positive for resolved sister telomeres whereas metaphase cells carrying two sets of a green singlet were scored positive for unresolved sister telomeres. Approximately 100 metaphase cells were scored for each cell line in blind. (f) Chromosome-specific FISH using a TRITC-labelled Alagille probe (JAG1/D20S1091) in red in conjunction with a FITC-labelled subtelomeric specific probe (20qter; Cytocell) in green. DNA was stained with DAPI shown in blue. Original magnification X100. (g) Quantification of metaphase cells carrying the separated chromosome arms. Metaphase cells carrying two sets of a red doublet were scored positive for the separated chromosome arms. Approximately 100 metaphase cells were scored for each cell line in blind. (h) Quantification of micronuclei formation in TRF1-depleted HeLaII cells expressing various constructs as indicated. Scoring of each cell line was done in a blind manner. For each cell line, at least a total of 3,060 cells from three independent experiments were scored. Standard deviations derived from three independent experiments are indicated. ThePvalues were calculated using a Student's two-tailedt-test. Figure 8: Lack of phosphorylation at T371 leads to near complete blockage of the resolution of sister telomeres. ( a ) Dot blots of anti-Myc ChIPs. TRF1-depleted HeLaII cells, expressing various constructs as indicated, were treated with nocodazole before ChIP analysis. ( b ) Quantification of anti-Myc ChIPs. Standard deviations derived from three independent experiments are indicated. ( c ) Western analysis of Myc-tagged TRF1 expression. ( d ) Chromosome-specific FISH with a FITC-labelled subtelomere specific probe (16pter; Cytocell) in green. DNA was stained with DAPI shown in blue. Original magnification X100. ( e ) Quantification of metaphase cells carrying unresolved sister telomeres. Metaphase cells carrying two sets of a green doublet were scored positive for resolved sister telomeres whereas metaphase cells carrying two sets of a green singlet were scored positive for unresolved sister telomeres. Approximately 100 metaphase cells were scored for each cell line in blind. ( f ) Chromosome-specific FISH using a TRITC-labelled Alagille probe (JAG1/D20S1091) in red in conjunction with a FITC-labelled subtelomeric specific probe (20qter; Cytocell) in green. DNA was stained with DAPI shown in blue. Original magnification X100. ( g ) Quantification of metaphase cells carrying the separated chromosome arms. Metaphase cells carrying two sets of a red doublet were scored positive for the separated chromosome arms. Approximately 100 metaphase cells were scored for each cell line in blind. ( h ) Quantification of micronuclei formation in TRF1-depleted HeLaII cells expressing various constructs as indicated. Scoring of each cell line was done in a blind manner. For each cell line, at least a total of 3,060 cells from three independent experiments were scored. Standard deviations derived from three independent experiments are indicated. The P values were calculated using a Student's two-tailed t -test. Full size image Analysis of chromosome-specific fluorescence in situ hybridization (FISH) using fluorescein isothiocyanate (FITC)-conjugated subtelomeric probe 16pter showed that 95% of sister telomeres in TRF1-depleted cells expressing the vector alone were fully resolved, giving rise to two telomere signals seen in metaphase cells ( Fig. 8d,e ). Depletion of TRF1 had no effect on the resolution of sister telomeres ( Fig. 8e ). Similar to the vector alone, overexpression of wild-type TRF1 or the phosphomimic mutant TRF1-T371D did not affect the resolution of sister telomeres ( Fig. 8d,e ). Full resolution of 96 and 94% of sister telomeres was observed in TRF1-depleted cells expressing either wild-type TRF1 or TRF1-T371D, respectively ( Fig. 8e ). In contrast, 91% of sister telomeres remained associated in TRF1-depleted cells expressing the non-phosphorylatable mutant TRF1-T371A ( Fig. 8d,e ), giving rise to a single telomere signal seen in metaphase cells ( Fig. 8d ). The failure of TRF1-T371A to resolve sister telomeres was also observed with a FITC-conjugated subtelomeric probe 20qter ( Fig. 8f ). However, no defect in the ability of TRF1-T371A to separate chromosome arms was detected ( Fig. 8f,g ), suggesting that the T371A mutation specifically abrogates the ability of TRF1 to resolve sister telomeres. In addition to its defect in the resolution of sister telomeres, we also observed a 2.2-fold increase in the number of micronuclei in the cell line expressing TRF1-T371A compared with that in the cell line expressing wild-type TRF1 ( Fig. 8h ). Such increase likely contributed to mild apoptosis and slow growth detected in TRF1-depleted cells expressing TRF1-T371A ( Fig. 7g,h ). These results altogether suggest that T371 phosphorylation by Cdk1 is required for the resolution of sister telomeres in early mitosis and that the blockage in sister telomere resolution may lead to chromosome missegregation and impaired cell proliferation. It has been a long-standing question as to whether Cdk1, a key mediator of mitotic entry, has a role in the separation of sister chromatids. In this study, we have uncovered that Cdk1 regulates the separation of sister telomeres by controlling TRF1, a shelterin protein that is known to interact with SA1 (ref. 18 ). Our work raises an interesting question as to whether Cdk1 might regulate the separation of chromosome arms by modulating proteins that interact with cohesin proteins. Our finding that failure to resolve sister telomeres is associated with the induction of micronuclei formation as well as impaired cell proliferation suggests that sister telomere resolution may be crucial for chromosome segregation and cell growth. T371 of TRF1 undergoes Cdk1-dependent phoshorylation on mitotic entry, and this phosphorylation is removed in late mitosis to allow re-association of TRF1 with telomeres. Using multiple approaches including IF, ChIP, differential salt extraction of chromatin and in vitro gel-shift assays, we have demonstrated that T371 phosphorylation by Cdk1 negatively regulates TRF1 interaction with telomeric DNA, arguing against the previously suggested possibility that T371 phosphorylation by Cdk1 serves as a positive regulator of TRF1 binding to telomeric DNA [29] 29. The weak anti-pT371 staining in interphase cells is not sensitive to treatment with Cdk1 inhibitors ( Fig. 1h ), suggesting that cyclin-dependent kinase(s) might not be involved in T371 phosphorylation in interphase cells. Although T371 of TRF1 does not appear to be involved in telomere replication, the phosphorylation status of T371 is essential for telomere protection and the separation of sister telomeres. Persistent phosphorylation of T371 promotes loss of telomere heterochromatin and telomere-bound TRF1, leading to induction of telomere loss and the formation of sister telomere fusions. The lack of a significant accumulation of micronuclei in TRF1-T371D-expressing cells is unclear. It is possible that sister telomere fusions might have promoted micronuclei formation, but these micronuclei might have escaped detection due to the rapid cell death. On the other hand, the lack of T371 phosphorylation promotes TRF1 association with telomeres in early mitosis, resulting in near blockage of sister telomere resolution. Accumulation of telomere loss was also observed in cells expressing TRF1-T371A, and yet there was no loss of telomere heterochromatin, suggesting that TRF1-T371A-induced telomere loss might occur by a distinct pathway from that of TRF-T371D. These results further imply that telomere loss might arise from forced separation of unresolved sister telomeres. Knockout of TRF1 in either mouse embryonic fibroblasts or mouse embryonic stem cells results in the formation of telomere fusions, indicative of telomere de-protection [4] , [5] . The lack of a severe telomere de-protection phenotype in TRF1-depleted cells may be due to the fact that shRNA-mediated knockdown did not completely eliminate endogenous TRF1 ( Fig. 1b ). Perhaps, the residual amount of endogenous TRF1 was able to provide sufficient telomere protection needed to sustain cell growth in TRF1-depleted cells. TRF1-T371D promotes telomere uncapping only in TRF1-depleted cells but not in TRF1-proficient cells, indicative of it being a loss of function mutation. The level of TRF1-T371D expressed in TRF1-depleted cells was over tenfold higher than the residual amount of endogenous TRF1. Conceivably, the excess amount of TRF1-T371D might titrate away the residual amount of endogenous TRF1 in TRF1-depleted cells. Such titration may in part account for the difference in phenotypes between TRF1-depleted cells expressing TRF1-T371D and TRF1-depleted cells. Mutations at T371 do not affect TRF1 interaction with TIN2 or tankyrase 1 (M.M. and X.-D.Z, unpublished results). Collectively, these results suggest that phenotypes associated with either T371A or T371D are likely due to an altered association of TRF1 with telomeres. We observed a net loss of total TRF1 at telomeres in mitosis, which is probably caused by a combined effect of the sequestration of unbound TRF1 by Cdk1 and the release of telomere-bound TRF1 ( Supplementary Fig. S8 ). It has been shown that poly(ADP-ribosyl)ation by tankyrase 1 releases TRF1 from telomeres, rendering it susceptible to degradation [23] . Perhaps the release of TRF1 from telomeres by tankyrase 1, in conjunction with T371 phosphorylation, may in part lead to the net loss of total TRF1 at telomeres in early mitosis. TRF1 binding to telomeres is very dynamic and there is a high exchange rate between bound TRF1 and free TRF1 [34] . When not bound to telomeric DNA, TRF1 is susceptible to degradation [23] , [24] . Although phosphorylated (pT371)TRF1 is excluded from associating with chromatin, it is more stable than the total TRF1. Similarly, the phosphomimic mutant TRF1-T371D is more stable than both wild-type TRF1 and the non-phosphorylable mutant TRF1-T371A, despite the fact that it has an impaired affinity for telomeric DNA. These results led us to propose that T371 phosphorylation by Cdk1 may temporally safeguard the pool of unbound TRF1 from being degraded in early mitosis when the resolution of sister telomeres occurs. Such temporal safeguard may provide the pool of TRF1 needed to re-establish telomere protection once chromosomes are pulled apart in late mitosis ( Supplementary Fig. S8 ). Plasmids and antibodies The QuickChange site-directed mutagenesis kit (Strategene) was used to generate TRF1 mutants (T371A, T371D and R425V) and wild-type TRF1 carrying silent mutations and resistant to shTRF1 from pLPC-N-myc-TRF1. Wild-type TRF1 and TRF1 mutants (T371A and T371D) were then subcloned into either the retroviral vector pWZL-N-myc [35] or the bacterial expression vector pHis-Parallel-2 (ref. 36 ). The annealed oligonucleotides encoding shTRF1 (5′-GAATATTTGGTGATCCAAA-3′) were ligated into pRetroSuper vector [9] , giving rise to pRetroSuper-shTRF1. The BgI II– Xho I fragment containing telomeric DNA in pTH12 was replaced with a Bgl II— Xho I fragment containing non-telomeric DNA, giving rise to the pTH12-NT plasmid. Rabbit polyclonal anti-pT371 antibody was developed by Biosynthesis against a TRF1 peptide containing phosphorylated threonine 371 (VSKSQPV-pT-PEKHRARKR). Antibodies to TRF1, TRF2 and TIN2 were gifts from Titia de Lange, Rockefeller University. Commercially obtained antibodies included γ-H2AX (Upstate), H3K9m3 (Upstate), H3-pS10 (Cell Signaling) and anti-γ-tubulin (GTU88, Sigma). Cell culture and synchronization Cells were grown in DMEM medium with 10% fetal bovine serum for HeLaI.2.11, HeLaII, GM637, Phoenix cells and 15% fetal bovine serum for hTERT-RPE, supplemented with non-essential amino acids, glutamine, 100 U ml −1 penicillin and 0.1 mg ml −1 streptomycin. Retroviral gene delivery was carried out as described [37] , [38] . Cell synchronization at G1/S boundary was carried out as previously described [28] with modifications. HeLaI.2.11 cells were first arrested with thymidine (2 mM) for 14 h, followed by washing in PBS for three times and then released into refresh media for 11 h. Subsequently, cells were arrested again with 2 mM thymidine for 14 h and washed in PBS for three times before their release into fresh media for 0–16 h. For mitotic synchronization, HeLaI.2.11 cells were treated with 100 ng ml −1 nocodazole (Sigma) for 16 h. To inhibit Cdk1 activity in mitosis, either 20 μM Roscovitin (Sigma) or 2 μM CGP74541A (Sigma) was added to cell cultures in the last 2 hours of nocodazole treatment. For inhibition of DNA replication, cells were treated with aphidicolin (0.2 μM) for 16 h as previously described [8] . Differential salt extraction of chromatin Differential salt extraction of chromatin was performed as described [31] except that cells were treated with either DMSO or nocodazole for 16 h before proceeding with the extraction. Protein extracts were prepared essentially as described [28] , [35] , with the exceptions that extracts used for the detection of γ-H2AX and H3K9m3 were prepared by dissolving cell pellets directly in 2× Laemmli buffer. Immunoblotting and immunoprecipitation were carried out essentially as described [28] , [35] . Recombinant TRF1 proteins and in vitro kinase assays Production of 6×His-tagged TRF1 proteins was carried out essentially as described [9] . Induction of wild-type and mutant TRF1 proteins was carried out overnight with 0.1 mM isopropylthiogalactoside at room temperature. The cell pellet was resuspended in binding buffer (20 mM Tris–HCl [pH 7.9] and 500 mM NaCl) and then lysed by sonication. Following centrifugation, the supernatant was incubated with nickel-resin (Qiagen) for 2 h at 4 °C. The beads were washed three times with 60 mM imidazole and bound proteins were eluted with a buffer containing 1 M imidazole, 20 mM Tris–HCl pH 7.9 and 0.5 M NaCl. For Cdk1 kinase assays, two micrograms of His-tagged wild-type or mutant TRF1, pre-incubated with either DNA or no DNA, was incubated with 40 units of Cdk1-cyclin B (NEB, P6020) in the presence of γ- 32 P-ATP according to the manufacturer. For Plk1 kinase assays, two micrograms of either His-tagged wild-type TRF1 or β-Casein (Sigma) were incubated with Plk1 (Millipore) in the presence of γ- 32 P-ATP according to the manufacturer. The sequential kinase assays were performed essentially as described [29] . Two micrograms of His-tagged wild-type or mutant TRF1 were first incubated with or without Cdk1 (NEB) in the presence of cold 1 mM ATP, followed by addition of γ- 32 P-ATP in conjunction with either Plk1 (Millipore) or no Plk1. Chromatin immunoprecipitations Chromatin immunoprecipitations were carried out essentially as described [39] , [40] . Cells were treated with nocodazole (Sigma) or DMSO for 16 h before the treatment with 1% formaldehyde in PBS. For experiments involving the release of cells from a nocodazole arrest, cells were treated with DMSO or 1 μM okadaic acid for either 30 min or 90 min before addition of PBS-buffered 1% formaldehyde. Otherwise, cells were directly fixed with 1% formaldehyde in PBS for 1 h, followed by sonication (10 cycles of 20 s each, 50% duty and 5 output). For each ChIP, 200 μl cell lysate (equivalent to 2×10 6 cells) was used. For the total telomeric DNA, two aliquots of 50 μl supernatant (corresponding to one-quarter of the amount of lysate used for IP) were processed along with the IP samples at the step of reversing the crosslinks. Four-fifths of immunoprecipitated DNA was loaded on the dot blots whereas two inputs each containing 5% of total DNA were included to assess the consistency of loading. The average of the two input signals was used for quantification of telomeric DNA recovered. The ratio of the signal from each ChIP relative to the average signal from the two input lanes was multiplied by 5% (5% represents 5% of total DNA) and a factor of 1.25 (because four-fifths of the precipitated DNA was loaded for each ChIP), giving rise to the percentage of total telomeric DNA recovered from each ChIP. Detection of telomeric DNA was done with a radioactively labelled 800-bp TTAGGG repeat-containing fragment, as previously described [39] . Immunofluorescence and chromosome specific FISH Immunofluoresence was performed as described [9] , [28] , [38] except for that cover slips for scoring of anaphase bridges, and lagging chromosomes were stained directly with DAPI. Chromosome-specific FISH was carried out as described [21] with modifications. Cells were treated with 100 ng ml -1 nocodazole for 1 h, collected by shake-off and then fixed twice in 3:1 methanol acetic acid for 15 min each. On the following day, cells were dropped onto slides and dried overnight at RT. Slides were washed in PBS twice for 5 min each, followed by dehydration in a series of 70, 85 and 100% ethanol. The dried slides were denatured at 80 °C for 10 min and hybridized with either the FITC-labelled subtelomere specific probe (16pter; Cytocell) alone or a combination of both TRITC-labelled Alagille probe (JAG1/D20S1091) and FITC-labelled subtelomeric specific probe (20qter; Cytocell) at RT for 2 h in the dark according to the manufacturer's instruction. Slides were washed twice in 70% formamide and 10 mM Tris (pH 7.2) for 15 min. Following three-times wash in PBS for 5 min, slides were counter-stained with 0.2 μg per ml DAPI and embedded in 90% glycerol/10% PBS containing 1 mg per ml p -phenylenediamine (Sigma). All cell images were recorded on a Zeiss Axioplan 2 microscope with a Hammamatsu C4742-95 camera and processed in Open Lab. Metaphase chromosome spreads Metaphase chromosome spreads were essentially prepared as described [10] , [38] . TRF1-depleted HeLaII cells expressing various TRF1 alleles or the vector alone were arrested in nocodazole (0.1 μg ml -1 ) for 90 min. Following arrest, cells were collected by trypsinization, incubated for 7 min at 37 °C in 75 mM KCl, and fixed in freshly made methanol/glacial acidic acid (3:1). Cells were stored overnight at 4 °C, dropped onto slides and air-dried overnight in a chemical hood. FISH analysis on metaphase chromosome spreads was carried out essentially as described [38] , [41] . Slides with chromosome spreads were incubated with 0.5 μg ml -1 FITC-conjugated-(CCCTAA)3 PNA probe (Biosynthesis) for 2 h at room temperature. Following incubation, slides were washed, counter-stained with 0.2 μg ml -1 DAPI, and embedded in 90% glycerol/10% PBS containing 1 mg ml -1 p -phenylene diamine (Sigma). In vitro gel shift assays In vitro gel shift assays were done essentially as described [40] , [42] with an end-labelled 188-bp Bgl II– Xho I fragment from plasmid pTH12 (ref. 42 . Bacteria-derived recombinant wild-type or mutant TRF1 protein was incubated with the end-labelled DNA (1 ng) at room temperature for 20 min in a 20-μl reaction containing 20 mM HEPES-KOH (pH7.9), 150 mM KCl, 5% (v/v) glycerol, 4% (w/v) Ficoll, 1 mM EDTA, 0.1 mM MgCl 2 , 0.5 mM DTT, 500 ng sheared Escherichia coli DNA and 50 ng β-Casein. The DNA-protein complexes were fractionated on a 0.7% agarose gel run in 0.1× TBE (8.9 mM Tris–base, 8.9 mM boric acid and 0.2 mM EDTA) at 130 V for 1 h at room temperature. Gels were dried and exposed to PhosphorImager screens and the signals on the gels were quantified by ImageQuant analysis. The combined signal from three TRF1–DNA complexes was normalized to the total input signal in the corresponding lane to give the percentage of total DNA converted to TRF1–DNA complexes. Growth curve and TUNEL assays Growth curve was conducted as described [9] , [43] . For TRF1-depleted HeLaII cells expressing the vector, wild-type TRF1 or TRF1 mutants, 2×10 4 cells per well were seeded in duplicates onto 12-well plates and experiments were done in triplicates. Cells were counted every 3 days and media was changed every 4 days. Cells expressing wild-type TRF1 or the vector alone were split 1:16 on the ninth day after seeding whereas cells expressing TRF1-T371A were split 1:16 on the twelfth day after seeding. The TUNEL assays were performed using the In situ Cell Death Detection kit (Roche) according to the manufacturer's protocol. How to cite this article: McKerlie, M. & Zhu, X.-D. Cyclin B-dependent kinase 1 regulates human TRF1 to modulate the resolution of sister telomeres. Nat. Commun. 2:371 doi: 10.1038/ncomms1372 (2011).